TOPBP1 recruits TOP2A to ultra-fine anaphase bridges to aid in their resolution During mitosis, sister chromatids must be faithfully segregated to ensure that daughter cells receive one copy of each chromosome. However, following replication they often remain entangled. Topoisomerase IIα (TOP2A) has been proposed to resolve such entanglements, but the mechanisms governing TOP2A recruitment to these structures remain poorly understood. Here, we identify TOPBP1 as a novel interactor of TOP2A, and reveal that it is required for TOP2A recruitment to ultra-fine anaphase bridges (UFBs) in mitosis. The C-terminal region of TOPBP1 interacts with TOP2A, and TOPBP1 recruitment to UFBs requires its BRCT domain 5. Depletion of TOPBP1 leads to accumulation of UFBs, the majority of which arise from centromeric loci. Accordingly, expression of a TOPBP1 mutant that is defective in TOP2A binding phenocopies TOP2A depletion. These findings provide new mechanistic insights into how TOP2A promotes resolution of UFBs during mitosis, and highlights a pivotal role for TOPBP1 in this process. Faithful chromosome segregation is critical in preventing genome attrition during cell division. This is underscored by the fact that the mechanisms governing this process are highly conserved throughout evolution. However, DNA topology changes during replication and as a result replicated sister chromatids can remain entwined due to topological constrains, such as catenation. If not resolved properly, these entanglements persist during anaphase to form ‘DNA bridges’ between the separating DNA masses of each daughter cell. These bridges can be generally divided into two distinct classes based on their ability to be stained with conventional DNA dyes, that is, stainable ‘anaphase bridges’ or non-stainable ‘ultra-fine anaphase bridges’ (UFBs) [1] . UFBs were first identified as thread-like DNA strands between daughter DNA masses, generally not stained by conventional DNA dyes but coated with the Bloom syndrome helicase (BLM) protein, as observed by immunofluorescence analyses [1] . BLM is a member of the RecQ helicase family, and mutations in this gene result in Bloom syndrome, a condition characterized by cancer predisposition and developmental abnormalities [2] . Subsequently, the Polo-like kinase-interacting checkpoint helicase (PICH) was also shown to localize to these UFBs where it co-localizes with BLM [3] . It was also demonstrated that PICH binding to UFBs results from the DNA substrate undergoing tension and stretching [4] , and that PICH association to UFBs is required for BLM recruitment [5] . A subset of UFBs arise from common genomic fragile sites, which can be induced by replication stress, for example, treatment with aphidicolin [6] . They most likely result from sister chromatid interlinks generated by unresolved replication intermediates, and are characterized by the presence of the Fanconi Anaemia (FA) protein FANCD2 forming foci localizing at either end of the bridge [6] . In addition, γH2AX foci are detected at the extremities of these bridges as mitosis progresses, suggesting induction of a DNA damage response [6] . Recently, elegant work from two groups has shown that resolution of these structures is an active, MUS81–EME1-dependent process [7] , [8] . However, the majority of UFBs do not associate with the FA proteins, and the mechanism governing their resolution remains more enigmatic [9] . These UFBs originate mainly from centromeric loci in the genome, which suggests that they arise from unresolved DNA catenanes of fully replicated DNA strands present in anaphase [3] , [9] . They diminish in number upon progression through mitosis, and DNA double-strand breaks are not readily detectible in the daughter cells [9] . This suggests that they must be decatenated by the end of mitosis presumably by topoisomerases, most likely topoisomerase IIα (TOP2A), as TOP2A is the main enzyme involved in removal of DNA catenation in vertebrates. Accordingly, treatment with TOP2A-specific inhibitor, ICRF-193 or razoxane, which locks the enzyme in the so-called ‘closed-clamp’ form, preventing disjunction of catenated sister duplexes, leads to an increase in centromeric-associated UFBs (C-UFBs) [1] , [3] . Interestingly, cohesin persists at the centromere until anaphase onset and can act as a physical barrier to TOP2A, thus cohesin removal is also required for chromatid decatenation [10] . However, the mechanism of TOP2A recruitment to these structures or in fact, any role in their resolution is unclear and remains a key question in the field [9] . Topoisomerase IIβ-binding protein 1 (TOPBP1) was initially identified in a yeast two-hybrid screen for factors interacting with the C-terminal region of DNA topoisomerase-IIβ [11] . TOPBP1 is a large, highly conserved, BRCT-domain-containing protein, with a crucial role in promoting efficient initiation of DNA replication, as well as the cellular response to replicative stress [12] , [13] , [14] . TOPBP1 is also necessary for proper mitotic progression [15] and has recently been shown to localize to UFB-like structures in yeast and transformed chicken cell lines [16] . Here we identify TOPBP1 as a novel interactor of TOP2A that is required to promote the resolution of C-UFBs. We establish that this interaction is highly enriched in the G2/M phase of the cell cycle, requires the C-terminal region of TOPBP1 and is essential for efficient resolution of C-UFBs. On the basis of these findings, we propose that TOPBP1 recruits TOP2A to UFBs to aid resolution of DNA entanglements between sister chromatids, and this function could contribute to the role that these proteins play in the maintenance of genome stability. TOPBP1 is a novel TOP2A-interacting protein To understand the mechanism of TOP2A recruitment to UFBs, we undertook an unbiased proteomic approach to map TOP2A’s protein–protein interactions. To this end, we performed immunoprecipitation (IP) experiments followed by mass spectrometry (IP/MS) analysis of TOP2A-associated proteins from HEK293 cells enriched in G2/M phase. Among known interactors including TOP1 (ref. 17 ), XRCC5 (ref. 18 ), the FACT complex subunit SSRP1 (ref. 19 ), Aurora B kinase [20] , HDAC1 (ref. 21 ), DDX21 (ref. 19 ) and CDC5L [22] , we also identified TOPBP1 as a novel putative TOP2A-binding partner ( Fig. 1a ). Given that TOPBP1/Dpb11 has been recently shown to localize to UFBs, we set out to validate this interaction [16] . First, we immunoprecipitated green fluorescent protein (GFP)–TOPBP1 from nocodazole-treated or asynchronous U2OS cells stably expressing this fusion protein at a level similar to that of the endogenous protein ( Fig. 1b ). We could readily detect endogenous TOP2A by western blotting of GFP–TOPBP1 immunoprecipitates in G2/M enriched cells ( Fig. 1b ). Accordingly, endogenous TOPBP1 was detected in reciprocal GFP–TOP2A immunoprecipitates from cell extracts ( Fig. 1c ), thus confirming that the two proteins likely exist in the same complex in cells. Enrichment in G2/M phase in all cases was determined by fluorescence-activated cell sorting analysis ( Supplementary Fig. 1a ). Thus far, TOPBP1 localization to UFBs has been reported only in yeast Saccharomyces cerevisiae and the transformed avian B-lymphoblastoid cell line DT40 (ref. 16 ). Therefore, we decided to test whether this was also the case in human transformed and importantly, primary cells. We found by antibody staining and immunofluorescence microscopy that in U2OS cells undergoing mitosis, TOPBP1 protein localized to ‘thread-like’ structures forming a bridge linking the daughter DNA masses in anaphase and early telophase cells ( Fig. 1d ). To verify that these were indeed UFBs, we counterstained the cells with an antibody directed against BLM, a known marker of UFBs, where a subset of TOPBP1 bridges also stained for BLM on the same bridge ( Fig. 1e ). Next, we validated that this localization was not an antibody-based artefact by reproducing this observation in U2OS cells stably expressing GFP–TOPBP1 ( Supplementary Fig. 1b ). We also confirmed this observation in another human cell line (HeLa cells, Fig. 1f ) and importantly, in a human primary cell line (human dermal fibroblasts, Fig. 1g ). Taken together, these data support the notion that TOPBP1 plays an evolutionarily conserved role in sister chromatid disjunction, and importantly demonstrates that this localization is likely to represent a physiological process associated with normal cell division. Interestingly, TOPBP1 seemed to stain only a part of the bridge and its co-localization with BLM is rare ( Fig. 1e ). 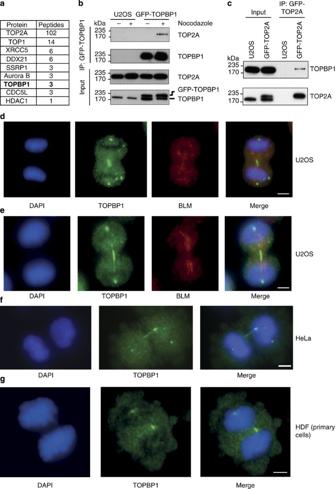Figure 1: TOPBP1 is a novel TOP2A-interacting protein that localizes to UFBs. (a) Proteins identified in IP/MS analysis of GFP-Trap purification from HEK 293FT cells expressing GFP–TOP2A. (b) Endogenous TOP2A co-immunoprecipitates with GFP-tagged TOPBP1. U2OS control cells or U2OS cells stably expressing GFP–TOPBP1 were untreated or treated with nocodazole (0.1 μg ml−1for 16 h) as indicated, and subjected to GFP-nanotrap immunoprecipitation. Input=0.4% of total IP. (c) Endogenous TOPBP1 co-immunoprecipitates with GFP-tagged TOP2A. U2OS control cells or U2OS cells stably expressing GFP–TOP2A were treated with nocodazole (0.1 μg ml−1for 16 h) and subjected to GFP-nanotrap immunoprecipitation. Input=0.4% of total IP. (d,e) Immunofluorescence microscopy in U2OS cells with antibodies against TOPBP1; BLM serves as a positive control. DAPI serves as a DNA stain. (f) Immunofluorescence microscopy of HeLa cells with antibodies against TOPBP1. DAPI serves as a DNA stain. (g) Immunofluorescence in human primary cells (human dermal fibroblasts) using antibody against TOPBP1. DAPI serves as a DNA stain. Scale bar, 6.4 μm. Figure 1: TOPBP1 is a novel TOP2A-interacting protein that localizes to UFBs. ( a ) Proteins identified in IP/MS analysis of GFP-Trap purification from HEK 293FT cells expressing GFP–TOP2A. ( b ) Endogenous TOP2A co-immunoprecipitates with GFP-tagged TOPBP1. U2OS control cells or U2OS cells stably expressing GFP–TOPBP1 were untreated or treated with nocodazole (0.1 μg ml −1 for 16 h) as indicated, and subjected to GFP-nanotrap immunoprecipitation. Input=0.4% of total IP. ( c ) Endogenous TOPBP1 co-immunoprecipitates with GFP-tagged TOP2A. U2OS control cells or U2OS cells stably expressing GFP–TOP2A were treated with nocodazole (0.1 μg ml −1 for 16 h) and subjected to GFP-nanotrap immunoprecipitation. Input=0.4% of total IP. ( d , e ) Immunofluorescence microscopy in U2OS cells with antibodies against TOPBP1; BLM serves as a positive control. DAPI serves as a DNA stain. ( f ) Immunofluorescence microscopy of HeLa cells with antibodies against TOPBP1. DAPI serves as a DNA stain. ( g ) Immunofluorescence in human primary cells (human dermal fibroblasts) using antibody against TOPBP1. DAPI serves as a DNA stain. Scale bar, 6.4 μm. Full size image TOPBP1 localization to UFBs is mediated via its BRCT 4 and 5 TOPBP1 carries out most of its functions via nine BRCT domains that mediate phosphorylation-dependent protein–protein interactions in several distinct complexes [23] . Importantly, only the BRCT domains 1/2 and 4/5 are conserved between yeast and human [24] . As TOPBP1’s yeast orthologue has been shown to localize to UFBs [16] , we hypothesized that these conserved BRCT domains may mediate its localization to UFBs in human cells. To test this, we generated pools of U2OS cells stably expressing GFP-tagged TOPBP1 BRCT1 and BRCT5 mutant proteins, with highly conserved lysine residues binding the phosphate group of the modified ligand, mutated to alanine ( Fig. 2a ), as we considered these domains as most likely to mediate TOPBP1’s interactions/recruitment [25] , [26] , [27] . We found that only the K704A TOPBP1 BRCT5 mutant protein was defective in its localization to UFBs in the absence of endogenous TOPBP1, with no defect observed for the GFP–TOPBP1 wild type (WT) or the GFP–TOPBP1 K154A-expressing cells ( Fig. 2b–d ; Supplementary Fig. 2a–c). To validate these data, we analysed single clones stably expressing the TOPBP1 mutant proteins. Again we found that only the BRCT domain-5 (K704A) mutant of TOPBP1 was defective in its localization to UFBs in the absence of endogenous TOPBP1, with no defect observed for the cells expressing GFP–TOPBP1 WT or GFP–TOPBP1 K154A ( Fig. 2e,f ; Supplementary Fig. 2d–f ). Moreover, and in support of the data above mutating the BRCT5 Lys704 to glutamic acid (K704E) also resulted in a profound defect in the ability of this mutant protein to localize to UFBs in the absence of endogenous TOPBP1 ( Fig. 2g ; Supplementary Fig. 2g ). In addition, given that BRCT domains interact with phosphorylated proteins, this suggested that a phosphorylated residue in a TOPBP1-interacting protein might mediate such localization. 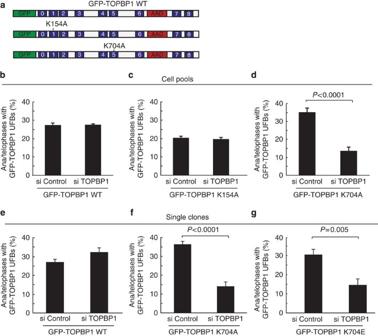Figure 2: BRCT5 of TOPBP1 mediates its recruitment to UFBs. (a) Schematic representation of GFP–TOPBP1 mutant constructs used in this study (WT TOPBP1, BRCT1—K154A; BRCT5—K704A). (b–d) Quantification of GFP–TOPBP1 WT, K154A and K704A mutant localization to UFBs in pools of U2OS cells stably expressing GFP–TOPBP1 WT or mutant proteins (endogenous TOPBP1 was knocked down using siRNA directed against the 3′ UTR (si TOPBP1); scrambled pool siRNA was used as a control (si Control)). Mean from three independent experiments is depicted with bars representing ±s.e.m. At least 50 ana/telophase cells were scored per experiment and theχ2-test was used to determine statistical significance. (e–g) Analysis of localization of GFP–TOPBP1 WT, K704A and K704E mutants to UFBs in single U2OS clones expressing GFP–TOPBP1 WT or mutant proteins (endogenous TOPBP1 was depleted using siRNA directed against the 3′ UTR (si TOPBP1); scrambled pool siRNA was used as a control (si Control)). Mean from three independent experiments is depicted with bars representing ±s.e.m. At least 50 ana/telophase cells were scored per experiment and theχ2-test was used to determine statistical significance. Figure 2: BRCT5 of TOPBP1 mediates its recruitment to UFBs. ( a ) Schematic representation of GFP–TOPBP1 mutant constructs used in this study (WT TOPBP1, BRCT1—K154A; BRCT5—K704A). ( b–d ) Quantification of GFP–TOPBP1 WT, K154A and K704A mutant localization to UFBs in pools of U2OS cells stably expressing GFP–TOPBP1 WT or mutant proteins (endogenous TOPBP1 was knocked down using siRNA directed against the 3′ UTR (si TOPBP1); scrambled pool siRNA was used as a control (si Control)). Mean from three independent experiments is depicted with bars representing ±s.e.m. At least 50 ana/telophase cells were scored per experiment and the χ 2 -test was used to determine statistical significance. ( e – g ) Analysis of localization of GFP–TOPBP1 WT, K704A and K704E mutants to UFBs in single U2OS clones expressing GFP–TOPBP1 WT or mutant proteins (endogenous TOPBP1 was depleted using siRNA directed against the 3′ UTR (si TOPBP1); scrambled pool siRNA was used as a control (si Control)). Mean from three independent experiments is depicted with bars representing ±s.e.m. At least 50 ana/telophase cells were scored per experiment and the χ 2 -test was used to determine statistical significance. Full size image BRCT5 of TOPBP1 mediates a phospho-dependent interaction between TOPBP1 and the BLM helicase, phosphorylated on Ser304 (ref. 28 ). Given the above and the fact that BLM localizes to UFBs, we considered the possibility that TOPBP1/BLM localization to these structures could be interdependent. To test this hypothesis, we analysed whether the BLM–TOPBP1 interaction was required to promote their recruitment to UFBs. However, BLM depletion had no discernable effect on the ability of TOPBP1 to localize to UFBs ( Supplementary Fig. 3a ), suggesting that BLM is not required for its recruitment to UFBs. BRCT domain 5 has been reported to mediate the interaction between TOPBP1 and MDC1, as well as 53BP1 (refs 29 , 30 ). Given that both these proteins associate with chromatin and promote TOPBP1 chromatin localization [29] , [30] , we considered the possibility that they may somehow promote TOPBP1 recruitment to UFBs. To test this, we knocked down MDC1 and 53BP1 and then analysed the kinetics of TOPBP1 recruitment to UFBs. We found that neither MDC1 nor 53BP1 knockdown had a major effect on TOPBP1 localization to UFBs ( Supplementary Fig. 3b,c ). Taken together, these data suggest that BLM, MDC1 and 53BP1 do not play a major role in TOPBP1 recruitment to UFBs. Finally, we also tested whether PICH depletion could result in deficient TOPBP1 localization to UFBs, as this protein is thought to be one of the first factors localizing to UFBs [5] . Again, knocking down PICH had no effect on TOPBP1 localization to UFBs, but as expected did cause a reduction in the incidence of BLM-positive UFBs ( Supplementary Fig. 3d,e ) [5] . In summary, this suggests that TOPBP1 localization to UFBs is most likely dependent on an as yet unidentified BRCT5-interacting protein. Given that TOPBP1 was identified on the basis of its association with the C terminus of TOP2B in a yeast two-hybrid screen, we considered the possibility that TOP2B may impact on the resolution of UFBs. To this end, we depleted TOP2B in U2OS cells and analysed the frequency of TOPBP1 and BLM UFBs. In line with TOP2B being non-essential for decatenation of DNA and progression through mitosis [31] , [32] , we found no significant change in the frequency of either type of UFBs ( Supplementary Fig. 3f–h ). The majority of TOPBP1-coated UFBs arise from centromeres UFBs can arise as a result of either decatenation or replication problems [1] , [9] . Given that we identify TOPBP1 as a novel TOP2A interactor, and that inhibition of TOP2A leads to an increase in C-UFBs [3] , [9] , we hypothesized that TOPBP1 may localize to this subtype of UFBs. To test this, we analysed the frequency of TOPBP1-coated UFBs in cells treated with aphidicolin, a potent DNA replication inhibitor, and razoxane, a specific topoisomerase II inhibitor [3] , [9] . Upon treatment with razoxane, but not aphidicolin, we could detect an increase in the percentage of ana/telophase cells with TOPBP1 UFBs ( Fig. 3a,b ). As an additional control to validate the efficacy of aphidicolin and razoxane treatment, we analysed the incidence of BLM UFBs under these experimental conditions. In line with previous reports and in support of the notion above, we observed a significant increase in BLM-positive UFBs upon drug treatment ( Fig. 3c ; Supplementary Fig. 4a,b ) [3] , [9] . Moreover, treatment with another TOP2A inhibitor ICRF-193 also resulted in an increased frequency of TOPBP1 UFBs with a concomitant increase in BLM UFBs ( Supplementary Fig. 4c,d ). This suggests that TOPBP1 is specifically recruited to UFBs arising as an effect of TOP2A inhibition. Moreover, the amount of TOPBP1 UFBs co-staining with BLM also increased following razoxane, but not with aphidicolin treatment ( Supplementary Fig. 4e,f ). TOP2A depletion and/or inhibition specifically increases the frequency of C-UFBs [1] , [3] , therefore if our hypothesis was correct then depletion of TOP2A should also result in an increased frequency of TOPBP1 UFBs, and indeed this is exactly what we observed ( Fig. 3d ; Supplementary Fig. 4g ). Importantly, this was also accompanied by an increase in BLM UFBs as well as 4',6-diamidino-2-phenylindole (DAPI)-positive anaphase bridges ( Fig. 3e,f ), a previously characterized phenotype of TOP2A deficiency [3] , [9] , [16] . Since treatment with the replication inhibitor aphidicolin did not increase the frequency of TOPBP1 UFBs but TOP2A depletion or inhibition did, these data suggest that TOPBP1 predominately associates with UFBs arising from centromeric loci (C-UFBs). These are most likely derived from problems associated with decatenation of sister chromatids and would require TOP2A for their resolution. 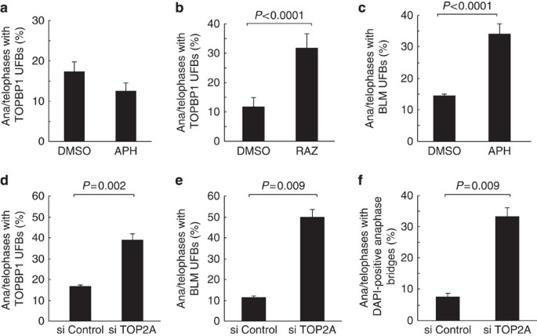Figure 3: TOP2A inhibition or depletion results in increased TOPBP1 localization to UFBs. (a,b) Quantification of the percentage of ana/telophase cells staining positive for TOPBP1 localization to UFBs in U2OS cells treated for 24 h with dimethylsulphoxide (DMSO) as a control, or with 0.4 μM aphidicolin (APH) or 10 μM razoxane (RAZ). Bars represent mean values from three independent experiments ±s.e.m. At least 50 ana/telophase cells were scored per experiment and theχ2-test was used to determine statistical significance. (c) Quantification of the percentage of U2OS ana/telophase cells staining positive for BLM UFBs in cells treated for 24 h with DMSO as a control or with 0.4 μM APH. Bars represent mean values from three independent experiments ±s.e.m. A minimum of 50 ana/telophase cells were scored per experiment, theχ2-test was used to determine statistical significance. (d) Quantification of the percentage of U2OS cells positive for TOPBP1 UFBs in cells treated with siRNA targeting TOP2A or in control siRNA-treated cells. Mean from three independent experiments with bars indicating ±s.e.m. At least 50 ana/telophase cells were scored per experiment, theχ2-test was used to determine statistical significance. (e,f) Quantification of the percentage of U2OS cells positive for BLM UFBs and DAPI-positive anaphase bridges, respectively. Cells were treated with siRNA directed against TOP2A or control siRNA. Mean from three independent experiments with bars indicating ±s.e.m. At least 50 ana/telophase cells were scored per experiment; theχ2-test was used to determine statistical significance. Figure 3: TOP2A inhibition or depletion results in increased TOPBP1 localization to UFBs. ( a , b ) Quantification of the percentage of ana/telophase cells staining positive for TOPBP1 localization to UFBs in U2OS cells treated for 24 h with dimethylsulphoxide (DMSO) as a control, or with 0.4 μM aphidicolin (APH) or 10 μM razoxane (RAZ). Bars represent mean values from three independent experiments ±s.e.m. At least 50 ana/telophase cells were scored per experiment and the χ 2 -test was used to determine statistical significance. ( c ) Quantification of the percentage of U2OS ana/telophase cells staining positive for BLM UFBs in cells treated for 24 h with DMSO as a control or with 0.4 μM APH. Bars represent mean values from three independent experiments ±s.e.m. A minimum of 50 ana/telophase cells were scored per experiment, the χ 2 -test was used to determine statistical significance. ( d ) Quantification of the percentage of U2OS cells positive for TOPBP1 UFBs in cells treated with siRNA targeting TOP2A or in control siRNA-treated cells. Mean from three independent experiments with bars indicating ±s.e.m. At least 50 ana/telophase cells were scored per experiment, the χ 2 -test was used to determine statistical significance. ( e , f ) Quantification of the percentage of U2OS cells positive for BLM UFBs and DAPI-positive anaphase bridges, respectively. Cells were treated with siRNA directed against TOP2A or control siRNA. Mean from three independent experiments with bars indicating ±s.e.m. At least 50 ana/telophase cells were scored per experiment; the χ 2 -test was used to determine statistical significance. Full size image To further explore the role of TOPBP1 in promoting resolution of C-UFBs, it was important to establish the consequences of TOPBP1 depletion on their resolution. To this end, we depleted TOPBP1 by short interfering RNA (siRNA) and analysed the frequency of BLM-positive UFBs. Upon TOPBP1 depletion, we detected a significant increase in the number of cells with BLM UFBs ( Fig. 4a ). One prediction from this notion would be that the TOPBP1 mutant defective in its association with UFBs (BRCT5 mutant) should display the same phenotype. In line with this, we detected a statistically significant increase in the number of BLM-positive UFBs in cells expressing this mutant protein, while cells expressing WT GFP–TOPBP1 (in the absence of endogenous TOPBP1) show no such increase under the same conditions ( Fig. 4a ), further validating the functionality of this fusion protein. Next, we addressed whether a physical link between these induced UFBs and centromeric DNA can be established. To do so, we stained cells for BLM and a centromeric marker, CENPB. Strikingly, the majority of the UFBs induced in the absence of TOPBP1 stained positive for CENPB ( Fig. 4b,c ), thus supporting the idea that TOPBP1 associates predominately with C-UFBs. Taken together, these data support a role for TOPBP1 in promoting chromosome disjunction by aiding resolution of C-UFBs. Moreover, BLM recruitment to UFBs seems to be TOPBP1-independent. 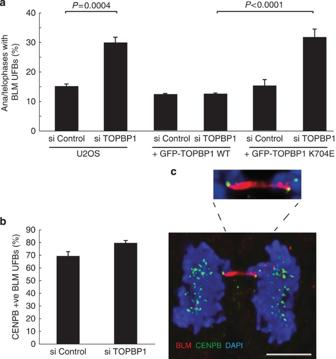Figure 4: TOPBP1 depletion impedes C-UFBs resolution. (a) Quantification of BLM-positive UFBs in control U2OS cells or cells stably expressing GFP–TOPBP1 WT or GFP–TOPBP1 K704E, respectively, in the presence or absence of endogenous TOPBP1. Mean from three independent experiments with bars indicating ±s.e.m. A minimum of 50 ana/telophase cells were scored per experiment and theχ2-test was used to determine statistical significance. (b) Quantification of UFBs emanating from centromeric loci, as assayed by CENPB staining in TOPBP1-depleted cells. Mean from three independent experiments with bars indicating ±s.e.m. A minimum of 50 ana/telophase cells were scored per experiment. (c) Representative image of an anaphase cell with a BLM-positive UFB (red) that emanates from a CENPB focus (green). DAPI (blue) serves as a DNA stain. Scale bar, 6.4 μm. Figure 4: TOPBP1 depletion impedes C-UFBs resolution. ( a ) Quantification of BLM-positive UFBs in control U2OS cells or cells stably expressing GFP–TOPBP1 WT or GFP–TOPBP1 K704E, respectively, in the presence or absence of endogenous TOPBP1. Mean from three independent experiments with bars indicating ±s.e.m. A minimum of 50 ana/telophase cells were scored per experiment and the χ 2 -test was used to determine statistical significance. ( b ) Quantification of UFBs emanating from centromeric loci, as assayed by CENPB staining in TOPBP1-depleted cells. Mean from three independent experiments with bars indicating ±s.e.m. A minimum of 50 ana/telophase cells were scored per experiment. ( c ) Representative image of an anaphase cell with a BLM-positive UFB (red) that emanates from a CENPB focus (green). DAPI (blue) serves as a DNA stain. Scale bar, 6.4 μm. Full size image TOPBP1 interacts with TOP2A via its C terminus To gain further insight into the potential functional relevance of the TOPBP1–TOP2A interaction, we designed a series of GFP-tagged TOPBP1 truncation constructs that sequentially removed single or tandem BRCT domains ( Fig. 5a ). We confirmed the efficacy of this approach by assaying their ability to interact with previously reported TOPBP1-binding partners ( Supplementary Fig. 5a ). Significantly, a TOPBP1 truncation mutant lacking the ATR-activation domain as well as the BRCT7 and 8 domains displayed no detectable binding to the endogenous TOP2A ( Fig. 5b ). To further map the minimal binding region, we generated TOPBP1 construct lacking only BRCT7 and 8 and found that this mutant was also defective in its interaction with TOP2A ( Fig. 5c ; Supplementary Fig. 5b , BLM and FANCJ were used as internal controls for this construct). This suggests that the extreme C terminus of TOPBP1 mediates its interaction with TOP2A. 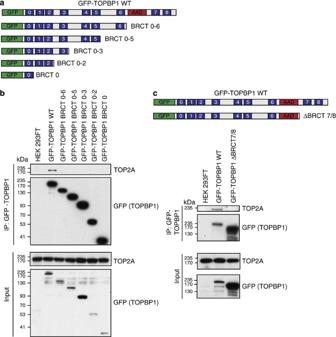Figure 5: TOPBP1–TOP2A interaction requires TOPBP1’s C terminus. (a) Schematic representation of GFP–TOPBP1 truncation mutants used inb. (b) TOPBP1–TOP2A interaction requires TOPBP1’s C terminus. HEK 293FT control cells, or cells transiently expressing WT GFP–TOPBP1 and indicated truncation mutants were nocodazole treated (0.1 μg ml−1for 16 h) and subjected to GFP-nanotrap immunoprecipitation. (c) TOPBP1–TOP2A interaction requires BRCT7/8. HEK 293FT control cells, or cells transiently expressing GFP–TOPBP1 WT or the indicated truncation mutant were nocodazole treated (0.1 μg ml−1for 16 h) and subjected to GFP-nanotrap immunoprecipitation. Figure 5: TOPBP1–TOP2A interaction requires TOPBP1’s C terminus. ( a ) Schematic representation of GFP–TOPBP1 truncation mutants used in b . ( b ) TOPBP1–TOP2A interaction requires TOPBP1’s C terminus. HEK 293FT control cells, or cells transiently expressing WT GFP–TOPBP1 and indicated truncation mutants were nocodazole treated (0.1 μg ml −1 for 16 h) and subjected to GFP-nanotrap immunoprecipitation. ( c ) TOPBP1–TOP2A interaction requires BRCT7/8. HEK 293FT control cells, or cells transiently expressing GFP–TOPBP1 WT or the indicated truncation mutant were nocodazole treated (0.1 μg ml −1 for 16 h) and subjected to GFP-nanotrap immunoprecipitation. Full size image Recently, both TOP2A and TOPBP1 have been reported to interact with components of the BRG1- or HRBM-associated factors (BAF) complex therefore, we tested whether BRG1 (the subunit of this complex that interacts with TOPBP1) promotes the TOP2A–TOPBP1 interaction [33] , [34] . However, knocking down BRG1 did not abrogate TOPBP1–TOP2A interaction ( Supplementary Fig. 6 ), suggesting that the two proteins interact directly or via another partner. TOPBP1 is required for TOP2A recruitment to UFBs Next, to address whether TOPBP1 promotes recruitment of TOP2A to UFBs to promote their decatenation, it was important to establish whether TOP2A and TOPBP1 co-localize on these structures. To this end, we optimized the recently developed proximity ligation assay (PLA) that allows the detection of protein–protein interactions at the single-molecule level by immunofluorescence microscopy [35] . Using this approach and employing antibodies directed against endogenous TOPBP1 and TOP2A, we were able to visualize co-localization of TOPBP1 and TOP2A on UFBs ( Fig. 6a,b ; Supplementary Fig. 7a ; these cells stably express GFP–TOPBP1, which serves as a marker of UFBs). Importantly, the majority of GFP–TOPBP1 UFBs observed were also associated with the PLA signal (co-localizing TOP2A–TOPBP1) ( Fig. 6c ). No PLA signal was observed in the negative control ( Fig. 6c ). Moreover, and in support of our hypothesis the TOPBP1 BRCT7/8 truncation mutant unable to bind TOP2A ( Fig. 5c ) showed defective co-localization of TOPBP1–TOP2A on UFBs, as assayed by the PLA technique ( Fig. 6d,e ). To our knowledge, this is the first time that TOP2A localization to UFBs has been observed. Given the above and the facts that (i) these two proteins co-immunoprecipitate in a cell enriched in the G2/M phase of the cell cycle and (ii) TOPBP1 depletion leads to the accumulation of C-UFBs, we hypothesized that TOPBP1 promotes recruitment of TOP2A to UFBs thereby aiding their resolution. 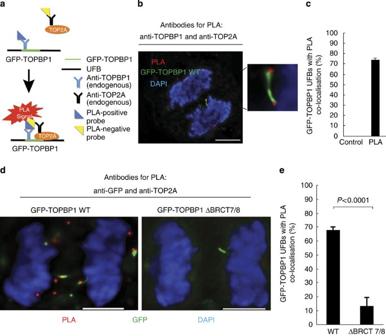Figure 6: TOP2A localizes to UFBs. (a) Schematic describing the proximity ligation assay (PLA) employed to visualize TOPBP1–TOP2A co-localization on UFBs. (b) Representative image of the PLA assay carried out using antibodies raised against endogenous TOPBP1 and TOP2A in U2OS cells stably expressing GFP–TOPBP1 WT. GFP acts as a marker for UFBs; PLA signal indicates TOPBP1–TOP2A co-localization. PLA signal co-localization with a UFB is highlighted in the zoomed section. Scale bar, 6.4 μm. (c) Quantification of the frequency of PLA co-localization with GFP–TOPBP1 UFBs. ‘Control’ represents the signal obtained for the PLA assay when using only one of the antibodies (TOP2A antibody). Mean from three independent experiments with bars indicating ±s.e.m. A minimum of 20 UFBs were scored per analysis. (d) Representative image of the PLA assay carried out using antibodies raised against GFP and TOP2A in U2OS cells transiently expressing GFP–TOPBP1 WT or BRCT7/8 truncation mutant. GFP acts as a marker for UFBs; PLA signal indicates TOPBP1–TOP2A co-localization. Scale bar, 6.4 μm. (e) Quantification of the frequency of PLA co-localization with GFP–TOPBP1 WT and BRCT7/8 truncation mutant. Mean from three independent experiments with bars indicating ±s.e.m. A minimum of 20 UFBs were scored per analysis and theχ2-test was used to determine statistical significance. Figure 6: TOP2A localizes to UFBs. ( a ) Schematic describing the proximity ligation assay (PLA) employed to visualize TOPBP1–TOP2A co-localization on UFBs. ( b ) Representative image of the PLA assay carried out using antibodies raised against endogenous TOPBP1 and TOP2A in U2OS cells stably expressing GFP–TOPBP1 WT. GFP acts as a marker for UFBs; PLA signal indicates TOPBP1–TOP2A co-localization. PLA signal co-localization with a UFB is highlighted in the zoomed section. Scale bar, 6.4 μm. ( c ) Quantification of the frequency of PLA co-localization with GFP–TOPBP1 UFBs. ‘Control’ represents the signal obtained for the PLA assay when using only one of the antibodies (TOP2A antibody). Mean from three independent experiments with bars indicating ±s.e.m. A minimum of 20 UFBs were scored per analysis. ( d ) Representative image of the PLA assay carried out using antibodies raised against GFP and TOP2A in U2OS cells transiently expressing GFP–TOPBP1 WT or BRCT7/8 truncation mutant. GFP acts as a marker for UFBs; PLA signal indicates TOPBP1–TOP2A co-localization. Scale bar, 6.4 μm. ( e ) Quantification of the frequency of PLA co-localization with GFP–TOPBP1 WT and BRCT7/8 truncation mutant. Mean from three independent experiments with bars indicating ±s.e.m. A minimum of 20 UFBs were scored per analysis and the χ 2 -test was used to determine statistical significance. Full size image If the above were correct then one would expect that cells expressing a mutant protein defective for TOPBP1–TOP2A interaction would display aberrant resolution of UFBs and increased incidence of DAPI-positive anaphase bridges, as observed in TOP2A-depleted cells ( Fig. 3e,f and ref. 36 ). We tested this hypothesis using TOPBP1 mutant defective in TOP2A interaction, but proficient in UFB localization ( Figs 5c and 6d ). In support of our line of thinking, cells expressing this TOPBP1 mutant protein phenocopied TOP2A depletion showing a significant increase in the incidence of both BLM UFBs as well as DAPI-positive anaphase bridges, as compared with mock-transfected control cells and cells expressing GFP–TOPBP1 WT ( Fig. 7a–c ). Moreover, the majority of these induced BLM UFBs emanated from centromeric loci, as assayed by CENPB staining ( Supplementary Fig. 7b ). Taken together, our data support a model whereby TOPBP1–TOP2A interaction promotes recruitment of TOP2A to centromeric UFBs to aid their resolution ( Fig. 7d ). 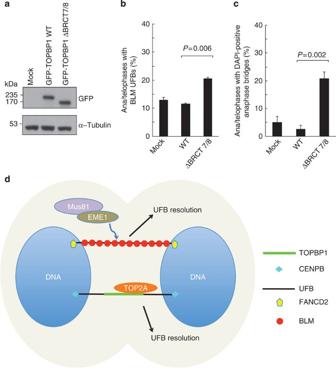Figure 7: TOPBP1–TOP2A interaction promotes UFB resolution. (a) Western blot depicting the levels of expression of GFP–TOPBP1 WT and GFP–TOPBP1 ΔBRCT7/8 mutant transiently expressed in U2OS cells (GFP). α-Tubulin serves as a loading control. (b,c) Quantification of the frequency of BLM UFBs or DAPI-positive anaphase bridges in mock-transfected U2OS cells (mock) or cells transiently expressing GFP–TOPBP1 WT or ΔBRCT7/8 mutant (WT or ΔBRCT7/8). Mean from three independent experiments with bars indicating ±s.e.m. A minimum of 50 ana/telophase cells were scored per experiment. Theχ2-test was used to evaluate statistical significance. (d) Schematic model of TOPBP1-mediated UFB resolution: TOPBP1 binds to C-UFBs via its BRCT5 domain and recruits TOP2A via its C terminus to aid their resolution. Figure 7: TOPBP1–TOP2A interaction promotes UFB resolution. ( a ) Western blot depicting the levels of expression of GFP–TOPBP1 WT and GFP–TOPBP1 ΔBRCT7/8 mutant transiently expressed in U2OS cells (GFP). α-Tubulin serves as a loading control. ( b , c ) Quantification of the frequency of BLM UFBs or DAPI-positive anaphase bridges in mock-transfected U2OS cells (mock) or cells transiently expressing GFP–TOPBP1 WT or ΔBRCT7/8 mutant (WT or ΔBRCT7/8). Mean from three independent experiments with bars indicating ±s.e.m. A minimum of 50 ana/telophase cells were scored per experiment. The χ 2 -test was used to evaluate statistical significance. ( d ) Schematic model of TOPBP1-mediated UFB resolution: TOPBP1 binds to C-UFBs via its BRCT5 domain and recruits TOP2A via its C terminus to aid their resolution. Full size image During every cell cycle DNA must be faithfully replicated and segregated to ensure that each daughter cell receives a copy of every chromosome. However, DNA topology changes during replication and as a result of this replicated sister chromatids remain entangled (catenated). The function of DNA catenation is not well understood but has been implicated in both sister chromatid cohesion and chromosome condensation [37] . What is clear, however, is the fact that for cells to undergo successful mitosis the DNA intertwining between sister chromatids needs to be completely removed. This process is thought to be regulated by DNA topoisomerase II type enzymes, and in particular TOP2A [31] , [32] . However, the experimental evidence for this as well as the possible mechanism governing TOP2A recruitment to UFBs remains enigmatic. In this study, we find that TOPBP1, a multifunctional replication/checkpoint protein, is a novel TOP2A interactor mediating its localization to UFBs originating from centromeric loci. To shed light on the mechanism of TOPBP1 recruitment to UFBs, we map the minimal region required for its localization to UFBs to BRCT motifs 4 and 5. Importantly, and in support of its role in UFBs’ resolution we show that depletion of TOPBP1, or mutation within the highly conserved lysine residue (K704) of the BRCT5, results in a sharp increase in the incidence of C-UFBs in the absence of endogenous TOPBP1. Replication inhibition increases the frequency of UFBs; however, the C-UFBs are thought not to contain aberrant DNA structures [36] . Since TOPBP1 depletion induces UFBs that primarily associate with the centromeric marker CENPB, we consider it unlikely that it is TOPBP1’s function in replication/checkpoint activation that drives this phenotype. This supports the idea that UFBs that require the action of TOPBP1 most likely originate from unresolved DNA catenanes that physically link sister chromatids, and have to be resolved before DNA segregation can take place. In support of this line of thinking, we show that treatment with TOP2A-specific inhibitors, but not DNA replication inhibitor aphidicolin, increases the number of TOPBP1-stained UFBs. Likewise, depletion of yeast TOP2 increases the frequency of DPB11/TOPBP1-coated UFBs, whereas aphidicolin treatment in both yeast as well as avian DT40 cells does not [16] . Moreover, C-UFBs generally are thought not to contain single-stranded DNA [36] , and in support of our hypothesis in chicken cells only a small proportion of TOPBP1 UFBs stain for RPA, a marker of single-stranded DNA [16] . Nevertheless, it is possible that TOPBP1 binds more than one type of bridge. However, we think that the majority that are stained with TOPBP1 are centromeric. Our in vivo mapping shows that TOPBP1 localization to UFBs requires its BRCT domain 5, and is most likely phospho-dependent. This is based on the fact that mutating Lys704, which directly contacts the phosphate group of the cognate binding partner [30] , [38] , to either alanine or glutamic acid abrogates TOPBP1 recruitment to UFBs. However, our data also show that none of the known TOPBP1 BRCT5-interacting proteins mediate its recruitment to UFBs. This is based on the observations that depletion of BLM, MDC1 or 53BP1 does not affect TOPBP1 recruitment to UFBs. Likewise, depleting TOPBP1 does not abrogate BLM recruitment. On the basis of the above, we conclude that TOPBP1 recruitment to UFBs is most likely independent of these proteins. This raises the question as to how TOPBP1 is being recruited to UFBs. TOPBP1 displays DNA-binding activity in vitro [39] therefore, it is possible that perhaps exposed DNA present within the UFBs acts as a substrate for TOPBP1 binding. Another possibility, which seems more likely, is that a phosphorylated residue on an as yet unidentified protein mediates this interaction. Interestingly, we noticed that a small proportion of BLM-positive bridges could be also stained for TOPBP1. Intriguingly, in the majority of such cases TOPBP1 stains only part of the bridge. It is unclear at present what would be the physiological relevance of this. It is tempting to hypothesize that TOPBP1 is recruited to promote resolution of centromeric DNA catenations early in mitosis, thereby promoting sister chromatid disjunction. Upon progression to anaphase, DNA entanglements that have not been resolved in a timely manner, may lead to formation of DNA bridges (which would be stained by TOPBP1). Subsequently, DNA tension would increase creating a substrate recognized by PICH, and this will allow for BLM loading on these structures [4] , [5] . TOPBP1 may promote decatenation of such structures, thus relieving the tension on the DNA strands. This in turn could result in dissociation of PICH and hence BLM, with TOPBP1 possibly remaining. This hypothesis is supported by the observation that the incidence of TOPBP1 on UFBs also staining for BLM is increased upon inhibition or depletion of TOP2A, and the fact that TOPBP1 recruitment to UFBs is BLM-independent. This could also account for the UFBs we observe staining positive for TOPBP1 but not BLM. Finally, in support of TOPBP1’s putative role in promoting recruitment of TOP2A to UFBs associated with centromeric loci, we not only determined that this interaction is highly enriched in G2/M phase, but also crucially visualize co-localization of TOPBP1 with TOP2A on UFBs. Moreover, expression of a TOPBP1 mutant no longer able to bind TOP2A resulted in a decrease in co-localization of TOP2A to TOPBP1 UFBs, as measured by the PLA technique. Moreover, it also led to a sharp increase in UFBs as well as DAPI-positive bridges and as such, it phenocopied TOP2A depletion. On the basis of the above findings, we propose the following possible mechanism for TOPBP1-dependent resolution of UFBs ( Fig. 7d ). TOPBP1 is recruited to UFBs via its intrinsic DNA-binding activity or by interaction with a phosphorylated amino acid from an as yet unidentified partner. This provides a binding platform for TOP2A recruitment to UFBs that is mediated via the C-terminal region of TOPBP1. This in turn promotes efficient TOP2A-dependent decatenation of sister chromatids before they are segregated during the final stages of mitosis. TOP2A is an essential enzyme with fundamental role in regulating DNA topology [40] . Overexpression/amplification of TOP2A is characteristic of many tumours and negatively correlates with patients’ survival [41] , [42] . This work provides an important molecular insight into the mechanism of TOPBP1–TOP2A interaction and resolution of the most prevalent class of UFBs (C-UFBs). Given that drugs targeting TOP2A, such as TOP2A poisons, are commonly used in anticancer treatment [43] , it is conceivable therefore, that the interaction described here could provide a framework for further studies aiming towards development of novel anticancer therapeutic approaches. Cell lines and chemicals HEK 293FT, HeLa and U2OS cells were a kind gift from Dr G. Stewart and Dr F. Esashi, respectively, and were cultured in DMEM containing 10% fetal bovine serum (FBS) and 1% of antibiotics solution (penicillin and streptomycin, Lonza) [44] . Primary dermal fibroblasts from neonatal human foreskin were purchased from CELLnTEC Advanced Cell Systems and cultured in MEM media supplemented with 10% FBS and 1% of antibiotics solution (penicillin and streptomycin, Lonza), as previously described [45] , [46] . Stable cell lines were generated by transfection with indicated constructs and maintained in media supplemented with 500 μg ml −1 G-418 followed by clonal selection. All chemicals were from Sigma-Aldrich, unless otherwise stated. SDS–PAGE and western blotting Primary antibodies and dilutions used in the outlined western blotting experiments were 53BP1 (MAB3802, Millipore, 1:3,000), α-tubulin (T5168, Sigma, 1:30,000), BLM (A300-110A, Bethyl Laboratories, 1:2,000), BRG1 (sc-10768, Santa Cruz Biotechnology, 1:200), FANCJ (B1310, Sigma, 1:5,000), GFP (11814460001, Roche, 1:1,000), MDC1 (obtained from Dr G. Stewart, University of Birmingham, 1:1,000 (ref. 47 )), PICH (04–1540, Millipore, 1:1,000), Rad9 (R7404, Sigma, 1:1,000), TOP2A (TG2011-1, Topogen, 1:1,000), TOP2B (ab58442, Abcam, 1:1,000) and TOPBP1 (A300-111A, Bethyl Laboratories, 1:5,000). SDS–PAGE and western blotting were performed as described previously [48] . Plasmids and transfections Plasmid construct encoding human GFP–TOPBP1 in pIRESneo2 (Clontech) vector backbone was obtained from Professor T.D. Halazonetis [30] . GFP–TOPBP1 truncation mutants or point mutants were generated by site-directed mutagenesis. Plasmid construct coding for human GFP–TOP2A in pEGFPC3 (Clontech) plasmid backbone [49] was obtained from Dr G.J. Gorbsky. GFP–TOP2A truncation mutants were generated by site-directed mutagenesis. Plasmids were transfected into human cells using Lipofectamine 2000 (Life Technologies), according to the manufacturer’s instructions. RNA interference treatment siRNAs targeting human 53BP1 (sc-37455) and BRG1 (sc-29827) and TOP2A (sc-36695) were obtained from Santa Cruz Biotechnology. siRNA pools targeting MDC1 (L-003506-00) and PICH (L-031581-01) were obtained from Dharmacon. Oligonucleotide mix targeting the 3′ untranslated region (UTR) of endogenous human TOPBP1 (Dharmacon) contained the following oligos: 5′-GUAAAUAUCUGAAGCUGUAUU-3′, 5′-GCACAAGGUUUAAUGAGGAUU-3′, 5′-GCUGUAGCUUAGUGGAAAUUU-3′. The oligonucleotide targeting the 3′ UTR of BLM (Dharmacon) was as follows: 5′-GCUAGGAGUCUGCGUGCGAUU-3′. siRNA targeting TOP2B was 5′-UCGGGCUAGGAAAGAAGUAAA-3′ (ref. 50 ): Santa Cruz Biotechnology non-targeting siRNA control (sc-37007) or Dharmacon non-targeting smart pool siRNA (D-00180-10-20) were used as control siRNAs where appropriate. Oligonucleotides were transfected into human cells using Oligofectamine reagent (Life Technologies), according to the manufacturer’s instructions. Co-immunoprecipitations For preparation of lysates for co-immunoprecipitations, cells were washed twice in phosphate-buffered saline and lysed in IP buffer (100 mM NaCl, 0.2% Igepal CA-630, 1 mM MgCl2, 10% glycerol, 5 mM NaF, 50 mM Tris-HCl, pH 7.5), supplemented with complete EDTA-free protease inhibitor cocktail (Roche) and 25 U ml −1 Benzonase (Novagen). After nuclease digestion, NaCl and EDTA concentrations were adjusted to 200 and 2 mM, respectively, and lysates were cleared by centrifugation (16,000 g for 25 min). Lysates were then incubated with 20 μl of GFP-Trap agarose beads (ChromoTek) for 2 h with end-to-end mixing at 4 °C. Complexes were washed extensively before resuspension in 2 × SDS sample buffer. Examples of full gel immunoblots from IP experiments are presented in Supplementary Figs 8 and 9 . For MS analyses, eluates from IP experiments were analysed by the Mass Spectrometry Laboratory (IBB PAS, Warsaw, Poland) using the Thermo Orbitrap Velos system, and protein hits were identified by MASCOT. Immunofluorescence microscopy Antibodies employed for immunofluorescence were as follows: BLM (sc-7790, Santa Cruz Biotechnology, 1:100), CENPB (ab25734, Abcam, 1:1,000), GFP (11814460001, Roche, 1:500 or 598, MBL, 1:500), TOP2A (MAB4197, Millipore, 1:1,000) and TOPBP1 (A300-111A, Bethyl Laboratories, 1:200). Mitotic cells were enriched by mitotic shake-off and centrifuged at 1,000 g for 3 min onto poly-L-Lysine slides (Thermo Scientific). Slides were fixed in 100% methanol for 20 min at −20 °C and blocked in 10% FBS in PBS for 30 min before incubation with indicated primary antibodies (in 0.1% FBS in PBS) for 1 h at room temperature. Unbound primary antibodies were removed by washing 4 × 5 min in PBS at room temperature followed by incubation with indicated secondary antibodies for 45 min at room temperature. Slides were then washed 4 × 5 min in PBS before mounting with Vectashield mounting medium (Vector Laboratories) with DAPI. For PLAs, antibodies against TOPBP1 (A300-111A, Bethyl Laboratories, 1:200) or GFP (598, MBL, 1:500) and TOP2A (MAB4197, Millipore, 1:1,000) were used with the Duolink In Situ Starter Kit (DUO92101-1KT, Sigma) according to the manufacturer’s recommendations. Images were acquired with a Zeiss Observer Z1 microscope using an X40 objective and ZEN 2012 (blue edition) software (Carl Zeiss). In some instances images were acquired with a DeltaVision DV Elite microscope using an X100 objective. Image analysis was carried out with FIJI (ImageJ) and Huygens Professional (Scientific Volume Imaging) software. Statistical analysis In all immunofluorescence experiments, a minimum of 50 ana/telophase cells per experiment were analysed in three independent experiments. The χ 2 -test was used to determine statistical significance, unless otherwise indicated in the figure legend. How to cite this article: Broderick, R. et al. TOPBP1 recruits TOP2A to ultra-fine anaphase bridges to aid in their resolution. Nat. Commun. 6:6572 doi: 10.1038/ncomms7572 (2015).